Dichotomy of the electronic structure and superconductivity between single-layer and double-layer FeSe/SrTiO3films The latest discovery of possible high-temperature superconductivity in the single-layer FeSe film grown on a SrTiO 3 substrate has generated much attention. Initial work found that, while the single-layer FeSe/SrTiO 3 film exhibits a clear signature of superconductivity, the double-layer film shows an insulating behaviour. Such a marked layer-dependent difference is surprising and the underlying origin remains unclear. Here we report a comparative angle-resolved photoemission study between the single-layer and double-layer FeSe/SrTiO 3 films annealed in vacuum. We find that, different from the single-layer FeSe/SrTiO 3 film, the double-layer FeSe/SrTiO 3 film is hard to get doped and remains in the semiconducting/insulating state under an extensive annealing condition. Such a behaviour originates from the much reduced doping efficiency in the bottom FeSe layer of the double-layer FeSe/SrTiO 3 film from the FeSe–SrTiO 3 interface. These observations provide key insights in understanding the doping mechanism and the origin of superconductivity in the FeSe/SrTiO 3 films. The FeSe superconductor is peculiar among the recently discovered iron-based superconductors [1] , [2] , [3] because it has the simplest crystal structure solely consisting of the FeSe layers that are believed to be one of the essential building blocks of the iron-based superconductors [4] . It also exhibits unique superconducting properties where the superconducting transition temperature ( T c ) can be markedly enhanced from ~8 K at ambient pressure to nearly 37 K under high pressure [5] . The latest indication of even higher T c ~80 K in the single-layer FeSe films grown on a SrTiO 3 substrate [6] , together with the observations of its unique electronic structure and nodeless superconducting gap [6] , [7] , [8] , [9] , has generated much interest [10] , [11] , [12] , [13] , [14] , [15] , [16] , [17] , [18] , [19] . Surprisingly, it was found from the scanning tunnelling microscopy (STM)/scanning tunnelling spectroscopy (STS) measurements that, on the given FeSe/SrTiO 3 film, while the single-layer film shows clear coherent peaks that are indicative of superconductivity, the double-layer film shows a semiconducting/insulating behaviour [6] . Such a disparate behaviour between the single-layer and double-layer FeSe/SrTiO 3 films is rather puzzling. In a conventional picture, superconductivity is usually suppressed with the decrease of the film thickness due to dimensionality effect and may disappear when the thickness gets to a few layers or one layer, as demonstrated by the Pb films grown on a silicon substrate [20] and the FeSe films grown on the graphene substrate [21] . Even if one assumes that superconductivity arises only from the interface between the bottom FeSe layer and the SrTiO 3 substrate, it remains hard to understand why the top FeSe layer does not become superconducting because of the proximity effect. It is thus significant to understand the electronic origin on the obvious disparity between the single-layer and double-layer FeSe/SrTiO 3 films. Understanding this difference is important to uncover the origin of superconductivity in the single-layer FeSe/SrTiO 3 film and may be helpful in further enhancing the superconducting temperature in the FeSe/SrTiO 3 films. In this paper, we report a comparative investigation between the single-layer and double-layer FeSe/SrTiO 3 films by carrying out a systematic angle-resolved photoemission study (ARPES) on the samples annealed in vacuum. We have uncovered distinct behaviours of the electronic structure and superconductivity between the single-layer and double-layer FeSe/SrTiO 3 films. We find that, like its single-layer FeSe/SrTiO 3 counterpart, the double-layer FeSe/SrTiO 3 film follows a similar tendency to transform from an initial N phase into an S phase when annealed in vacuum. But it is much harder for the double-layer FeSe/SrTiO 3 film to get doped in transforming completely from the N phase into the S phase and becoming superconducting. This difference lies in the much reduced doping efficiency in the bottom FeSe layer for the double-layer and multiple-layer FeSe/SrTiO 3 films. These observations provide key information in understanding the origin of superconductivity and the doping mechanism of the FeSe/SrTiO 3 films. They also point to a possibility to further enhance superconductivity in the double-layer and multiple-layer FeSe/SrTiO 3 films. Electronic structure of the double-layer FeSe/SrTiO 3 film The previous detailed ARPES measurements keeping track on the electronic structure evolution of the single-layer FeSe/SrTiO 3 film from the initial non-superconducting sample to the superconducting sample revealed that, the as-grown sample is mainly composed of the ‘N phase’ while the superconductivity appears in the ‘S phase’ with sufficient electron doping [8] , [22] . The N phase and S phase exhibit distinct electronic structures and they compete and coexist in the intermediate annealing process [8] . 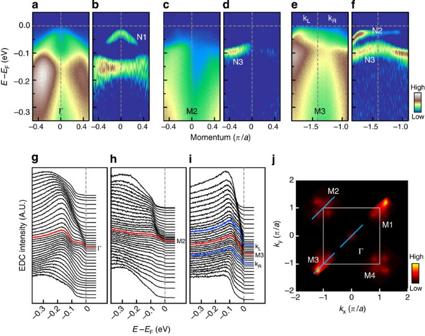Figure 1:  Electronic structure of the as-prepared double-layer FeSe/SrTiO3film. The data were taken on double-layer FeSe/SrTiO3film after the sample was annealed at 190 °C in vacuum for 1 h to remove the amorphous Se-capping layer. This sample contains the pure N phase. (a) Band structure along the cut 1 crossing the Γ point. Its corresponding second derivative image with respect to energy is shown inb. A hole-like band is observed labelled as N1. (c) Band structure for the cut 2 crossing the M2 point and its corresponding second derivative image is shown ind. (e) Band structure along the cut 3 crossing the M3 point with its corresponding second derivative image is shown inf. A hole-like band labelled as N2 is marked inf. It is strong on the left side, but weak on the right side possibly due to the photoemission matrix element effect. Another hole-like band N3 is also observed. (g–i) Photoemission spectra (energy distribution curves, EDCs) for the cut 1, cut 2 and cut 3, respectively. The EDCs at high symmetry points are marked in red, and the EDCs near the top of the N2 band are marked in blue. (j) Fermi surface of the as-prepared double-layer FeSe/SrTiO3film obtained by integrating the spectral weight near a small energy window (−0.03 eV,−0.01 eV) near the Fermi level. The three momentum cuts (cut 1, cut 2 and cut 3) are marked in the figure. For convenience, the four Brillouin zone corners are labelled as M1, M2, M3 and M4. Figure 1 shows the electronic structure of the as-prepared double-layer FeSe/SrTiO 3 film. The band structure around Γ ( Fig. 1a,b ) is characterized by a hole-like band denoted as N1 and another band at a higher binding energy. Its band structure across M3 ( Fig. 1e ) exhibits two hole-like bands at low temperatures, with one N2 band close to the Fermi level and the other N3 band nearly 70 meV below the Fermi level. The ‘Fermi surface’ ( Fig. 1j ) (here we use Fermi surface in a loose sense in that it corresponds to the maximum intensity contour in the spectral distribution in the momentum space) is characterized by four ‘strong spots’ around the M point and remnant weak spectral weight near the Γ point. These results are similar to that of the as-prepared single-layer FeSe/SrTiO 3 film that contains the pure N phase [8] . We have carefully examined the energy bands close to the Fermi level and found no indication of band crossing for these bands, including the N2 band ( Fig. 1g–i ). This indicates that the as-prepared double-layer FeSe/SrTiO 3 film is semiconducting/insulating, similar to the N phase of the as-prepared single-layer FeSe/SrTiO 3 film [8] . Figure 1:  Electronic structure of the as-prepared double-layer FeSe/SrTiO 3 film. The data were taken on double-layer FeSe/SrTiO 3 film after the sample was annealed at 190 °C in vacuum for 1 h to remove the amorphous Se-capping layer. This sample contains the pure N phase. ( a ) Band structure along the cut 1 crossing the Γ point. Its corresponding second derivative image with respect to energy is shown in b . A hole-like band is observed labelled as N1. ( c ) Band structure for the cut 2 crossing the M2 point and its corresponding second derivative image is shown in d . ( e ) Band structure along the cut 3 crossing the M3 point with its corresponding second derivative image is shown in f . A hole-like band labelled as N2 is marked in f . It is strong on the left side, but weak on the right side possibly due to the photoemission matrix element effect. Another hole-like band N3 is also observed. ( g – i ) Photoemission spectra (energy distribution curves, EDCs) for the cut 1, cut 2 and cut 3, respectively. The EDCs at high symmetry points are marked in red, and the EDCs near the top of the N2 band are marked in blue. ( j ) Fermi surface of the as-prepared double-layer FeSe/SrTiO 3 film obtained by integrating the spectral weight near a small energy window (−0.03 eV,−0.01 eV) near the Fermi level. The three momentum cuts (cut 1, cut 2 and cut 3) are marked in the figure. For convenience, the four Brillouin zone corners are labelled as M1, M2, M3 and M4. 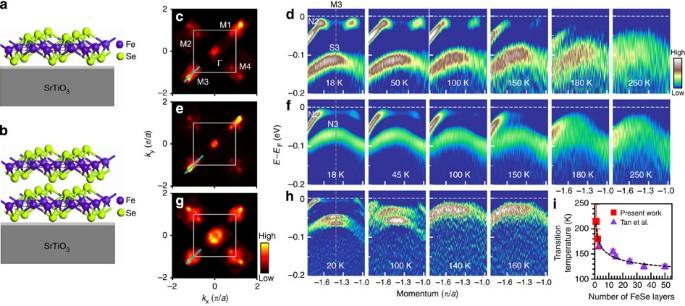Figure 2: Temperature dependence of the electronic structure for the single-layer and double-layer FeSe/SrTiO3films and BaFe2As2. (a,b) schematic structure of single-layer and double-layer FeSe films grown on SrTiO3(001) substrate, respectively. (c) Fermi surface of the single-layer FeSe/SrTiO3film measured at 18 K obtained by integrating the spectral weight over a small energy window (−0.03 eV,−0.01 eV). (d) Temperature dependence of the band structure measured along the M3 cut as shown incfor the single-layer FeSe/SrTiO3film. Owing to preparation condition variation, this as-prepared sample contains mainly the N phase as indicated by the strong N2 band and the S phase that is indicated by the S3 band. The sample status is similar to the sequence 7 in ref.8. The band structures shown here, as well as those infandh, are the second derivatives of the original bands with respect to the energy, to highlight the bands better8. One can see that the hole-like band N2, which is obvious at low temperatures, get weaker with increasing temperature and becomes invisible at 250 K. (e) Fermi surface of the as-prepared double-layer FeSe films measured at 18 K. (d) Temperature dependence of the band structure measured along the M3 cut as shown ine. The hole-like band N2 disappears at ~180 K. (g) Fermi surface of BaFe2As2measured at 40 K, which is below the magnetic transition temperature at ~138 K (ref.23). (h) Temperature dependence of its band structure across the M3 point23. (i) The transition temperature as a function of the number of FeSe layers in the FeSe/SrTiO3films. Here the transition temperature for the single-layer and double-layer FeSe/SrTiO3films (red squares) is determined from the temperature dependence of the band structure (d,f) where the hole-like N2 bands begin to disappear. The temperature for other films (violet triangles) with more FeSe layers is taken from Tanet al.9 Full size image Figure 2 shows the Fermi surface and the temperature dependence of the band structure across the M3 cut for the single-layer FeSe/SrTiO 3 film ( Fig. 2d ), the as-prepared double-layer FeSe/SrTiO 3 film ( Fig. 2f ) and BaFe 2 As 2 ( Fig. 2h ) [23] . Owing to preparation condition variation, the single-layer FeSe/SrTiO 3 film measured here contains mainly the N phase as indicated by the characteristic N2 band ( Fig. 2d ). It also contains the S phase that is indicated by the S3 band (the status of the sample is similar to the sequence 7 in ref. 8 ). With increasing temperature, the N2 band gets weaker, lowering down in its energy position, and becomes invisible at 250 K. The as-prepared double-layer FeSe/SrTiO 3 film shows rather similar temperature dependence of its electronic behaviour ( Fig. 2f ) as that of the single-layer FeSe film. In this case, the N2 band gets weaker with the increasing temperature and nearly disappears at 180 K. It appears that, with increasing temperature, the N2 band gradually merges into the N3 band and eventually becomes only one band above a transition temperature. As seen from Fig. 2 , the electronic structure of the as-prepared single-layer and double-layer FeSe/SrTiO 3 films shows a clear resemblance to that of the parent compound BaFe 2 As 2 in its magnetic state ( Fig. 1g,h ) [23] , in terms of the Fermi surface near the M point, the band structure near the M point and its temperature dependence. They are also very similar to that of the multiple-layer FeSe/SrTiO 3 films [9] . These observations suggest a possibility that the N phase in the as-prepared single-layer and double-layer FeSe/SrTiO 3 films is likely magnetic, as indicated before [8] , [9] . The present observation of the N phase in the double-layer FeSe/SrTiO 3 film, together with our previous observation of the N phase in the single-layer FeSe/SrTiO 3 film [8] and its observation in the triple- and multiple-layer FeSe/SrTiO 3 films [9] , has established a unified picture for its universal existence in the FeSe/SrTiO 3 films. The transition temperature of the N phase in the single-layer and double-layer FeSe/SrTiO 3 films, determined from the temperature dependence of the band structure across M3 where the N2 band starts to disappear ( Fig. 1d,f ), is shown in Fig. 1i , together with the temperature for the multiple-layer FeSe/SrTiO 3 films [9] . It follows the similar trend found for the multiple-layer FeSe/SrTiO 3 films [9] , such as, it decreases with the increasing number of the FeSe layers. The single-layer and double-layer FeSe/SrTiO 3 films are peculiar in that their N phase exhibits the highest transition temperature among all the FeSe/SrTiO 3 films. Figure 2: Temperature dependence of the electronic structure for the single-layer and double-layer FeSe/SrTiO 3 films and BaFe 2 As 2 . ( a , b ) schematic structure of single-layer and double-layer FeSe films grown on SrTiO 3 (001) substrate, respectively. ( c ) Fermi surface of the single-layer FeSe/SrTiO 3 film measured at 18 K obtained by integrating the spectral weight over a small energy window (−0.03 eV,−0.01 eV). ( d ) Temperature dependence of the band structure measured along the M3 cut as shown in c for the single-layer FeSe/SrTiO 3 film. Owing to preparation condition variation, this as-prepared sample contains mainly the N phase as indicated by the strong N2 band and the S phase that is indicated by the S3 band. The sample status is similar to the sequence 7 in ref. 8 . The band structures shown here, as well as those in f and h , are the second derivatives of the original bands with respect to the energy, to highlight the bands better [8] . One can see that the hole-like band N2, which is obvious at low temperatures, get weaker with increasing temperature and becomes invisible at 250 K. ( e ) Fermi surface of the as-prepared double-layer FeSe films measured at 18 K. ( d ) Temperature dependence of the band structure measured along the M3 cut as shown in e . The hole-like band N2 disappears at ~180 K. ( g ) Fermi surface of BaFe 2 As 2 measured at 40 K, which is below the magnetic transition temperature at ~138 K (ref. 23 ). ( h ) Temperature dependence of its band structure across the M3 point [23] . ( i ) The transition temperature as a function of the number of FeSe layers in the FeSe/SrTiO 3 films. Here the transition temperature for the single-layer and double-layer FeSe/SrTiO 3 films (red squares) is determined from the temperature dependence of the band structure ( d , f ) where the hole-like N2 bands begin to disappear. The temperature for other films (violet triangles) with more FeSe layers is taken from Tan et al. [9] Full size image Difference between single-layer and double-layer FeSe/SrTiO 3 films The distinct behaviours between the single-layer and double-layer FeSe/SrTiO 3 films show up when the as-prepared samples are post-annealed in vacuum under a similar condition. It was shown before that the as-prepared single-layer FeSe/SrTiO 3 film, after annealing in vacuum, can transform completely from a pure N phase into a pure S phase [8] , with its Fermi surface and band structure along typical momentum cuts shown in Fig. 3 (corresponding to the annealing sequence 10 in ref. 8 ). The Fermi surface of the S phase single-layer FeSe/SrTiO 3 film ( Fig. 3a ) is characterized by an electron-like Fermi surface around the M points while there is no indication of the Fermi surface near the Γ point [7] , [8] . Its corresponding band structure near Γ point shows a hole-like band with its top nearly 80 meV below the Fermi level ( Fig. 3b ) and there is an electron-like band crossing the Fermi level near M ( Fig. 3c,d ) [7] . For this particular annealed single-layer FeSe/SrTiO 3 film, it shows a superconducting gap that closes near 40 K (ref. 8 ). However, under an identical annealing condition, the double-layer FeSe/SrTiO 3 film remains in the N phase, with its Fermi surface ( Fig. 3e ) and band structure ( Fig. 3f–h ) similar to those of the as-prepared double-layer FeSe/SrTiO 3 film. This result is consistent with the previous STM observation that, in the same FeSe/SrTiO 3 film, while the single-layer area shows a superconducting coherence peak with its position at 20.1 meV, the double-layer area shows a semiconducting/insulating behaviour [6] . Both the present ARPES results and previous STM results [6] indicate that the double-layer FeSe/SrTiO 3 film indeed behaves quite differently from its single-layer counterpart, if prepared and annealed under similar conditions. 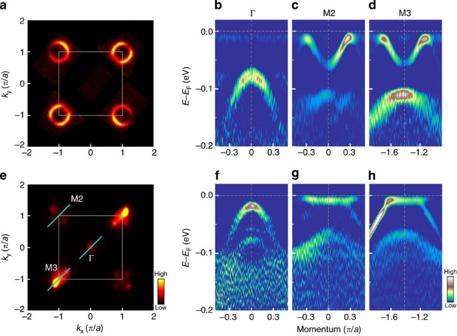Figure 3:  Dichotomy of the electronic structure between the single-layer and double-layer FeSe/SrTiO3films. The annealing condition corresponds to the sequence 10 in ref.8. (a) Fermi surface of the annealed single-layer FeSe/SrTiO3film. (b–d) Corresponding band structure of the annealed single-layer FeSe/SrTiO3film along the Γ, M2 and M3 cuts, respectively. (e) Fermi surface of the annealed double-layer FeSe/SrTiO3film. (f–h) Corresponding band structure of the annealed double-layer FeSe/SrTiO3film along the Γ, M2 and M3 cuts, respectively. The band structures shown in (b–d) and (f–h) are second derivatives of the original band with respect to energy. Figure 3:  Dichotomy of the electronic structure between the single-layer and double-layer FeSe/SrTiO 3 films. The annealing condition corresponds to the sequence 10 in ref. 8 . ( a ) Fermi surface of the annealed single-layer FeSe/SrTiO 3 film. ( b – d ) Corresponding band structure of the annealed single-layer FeSe/SrTiO 3 film along the Γ, M2 and M3 cuts, respectively. ( e ) Fermi surface of the annealed double-layer FeSe/SrTiO 3 film. ( f – h ) Corresponding band structure of the annealed double-layer FeSe/SrTiO 3 film along the Γ, M2 and M3 cuts, respectively. The band structures shown in ( b – d ) and ( f – h ) are second derivatives of the original band with respect to energy. Full size image Vacuum annealing of the double-layer FeSe/SrTiO 3 films One immediate question arising is whether one can transform the double-layer FeSe/SrTiO 3 film into the S phase, and even make it superconducting, by enhancing the annealing condition, as has been done for the single-layer FeSe/SrTiO 3 film [8] . The annealing condition can be enhanced in two ways: increasing the annealing time or elevating the annealing temperature. We used both ways to anneal the double-layer FeSe/SrTiO 3 film on two separate samples, and the results are shown in Fig. 4 (for the sample #1) and Fig. 5 (for the sample #2) (see Methods for the details of the annealing conditions). 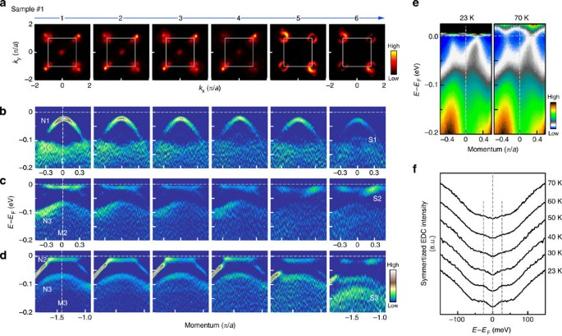Figure 4:  Electronic structure of double-layer FeSe/SrTiO3film (sample #1) annealed at 350 °C for different times. The sequences 1–6 correspond to an accumulative time of 15, 30.5, 46.5, 66.5, 87.5 and 92.5 h, respectively (see Methods for experimental details). (a) Fermi surface evolution as a function of the annealing time. (b–d) Band structure evolution with annealing time for the momentum cuts across Γ (b), M2 (c) and M3 (d). The location of the three cuts are the same as shown inFig. 3e. The band structures shown here are second derivatives of the original images with respect to energy. (e) Band structure (original data) of the annealed double-layer FeSe/SrTiO3film (corresponding to the sequence 6) along cut 2 across M2 measured at 23 K (left panel) and 70 K (right panel). The photoemission images are divided by the corresponding Fermi distribution function to highlight opening or closing of an energy gap. (f) Corresponding symmetrized EDCs on the Fermi momentum measured at different temperatures. Figure 4a shows the Fermi surface evolution of the double-layer FeSe/SrTiO 3 film (sample #1) with the increase of annealing time at a constant annealing temperature of 350 °C. The corresponding evolution of the band structure along three typical cuts is shown in Fig. 4b–d . With the increase of the annealing time, the initial N phase bands get weaker but are still present until the last annealing sequence 6, which already has a long annealing time over 90 h. New features corresponding to the S phase (S1, S2 and S3 bands marked in Fig. 4 ) start to appear in the sequence 5 and become clear for the sequence 6. During the annealing process, the double-layer FeSe/SrTiO 3 film undergoes a transition from the N phase into the S phase. This trend of evolution is rather similar to that observed in the single-layer FeSe/SrTiO 3 sample, but it corresponds to an early annealing stage where the major N phase coexists with the emergent minor S phase [8] . Figure 4e shows the band structure of the sample #1 across M2 at low (left panel) and high (right panel) temperatures for the last sequence 6. The Fermi distribution function is removed to highlight a possible gap opening near the Fermi level. The symmetrized energy distribution curves (EDCs) near the underlying Fermi momentum, measured at different temperatures, are shown in Fig. 4f . An energy gap of ~18 meV is observed at a low temperature of 23 K, which manifests itself as the appearance of a dip in the symmetrized EDCs ( Fig. 4f ) and a suppression of the spectral weight near the Fermi level in the photoemission image ( Fig. 4e ). The EDC peak is broad. The gap size shows little change with temperature and does not close until 70 K ( Fig. 4f,e ). All these observations indicate that the observed energy gap is an insulating gap. This is consistent with the case in the single-layer FeSe/SrTiO 3 film where it is found that, in the early annealing stage when the S phase just appears and has a low doping level, it opens an insulating gap [22] . Figure 4:  Electronic structure of double-layer FeSe/SrTiO 3 film (sample #1) annealed at 350 °C for different times. The sequences 1–6 correspond to an accumulative time of 15, 30.5, 46.5, 66.5, 87.5 and 92.5 h, respectively (see Methods for experimental details). ( a ) Fermi surface evolution as a function of the annealing time. ( b – d ) Band structure evolution with annealing time for the momentum cuts across Γ ( b ), M2 ( c ) and M3 ( d ). The location of the three cuts are the same as shown in Fig. 3e . The band structures shown here are second derivatives of the original images with respect to energy. ( e ) Band structure (original data) of the annealed double-layer FeSe/SrTiO 3 film (corresponding to the sequence 6) along cut 2 across M2 measured at 23 K (left panel) and 70 K (right panel). The photoemission images are divided by the corresponding Fermi distribution function to highlight opening or closing of an energy gap. ( f ) Corresponding symmetrized EDCs on the Fermi momentum measured at different temperatures. 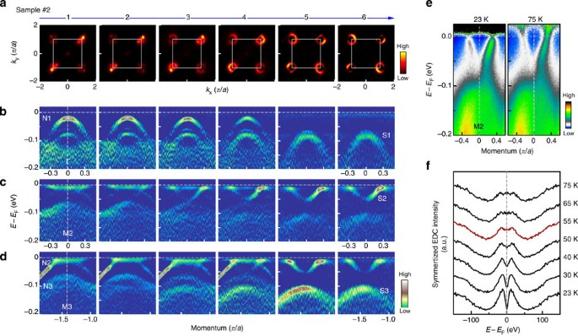Figure 5:  Electronic structure of the double-layer FeSe/SrTiO3film (sample #2) annealed with increasing temperatures. The highest annealing temperature is 350 °C for the sequence 1, 450 °C for the sequence 2, 500 °C for the sequence 3, 535 °C for the sequence 4 and then kept at 535 °C to increase the annealing time for the sequences 5 and 6. Refer to the Methods for experimental details of the annealing process. (a) Fermi surface evolution during the annealing process. (b–d) Band structure evolution for the momentum cuts across Γ (b), M2 (c) and M3 (d). The location of the three cuts are the same as shown inFig. 3e. The band structures shown here are second derivatives of the original images with respect to energy. (e) Band structure (original data) of the annealed double-layer FeSe/SrTiO3film (corresponding to the sequence 6) measured along cut 2 across M2 at 23 K (left panel) and 75 K (right panel). The photoemission images are divided by the corresponding Fermi distribution function to highlight opening or closing of an energy gap. (f) Corresponding symmetrized EDCs on the Fermi momentum measured at different temperatures. Full size image Figure 5:  Electronic structure of the double-layer FeSe/SrTiO 3 film (sample #2) annealed with increasing temperatures. The highest annealing temperature is 350 °C for the sequence 1, 450 °C for the sequence 2, 500 °C for the sequence 3, 535 °C for the sequence 4 and then kept at 535 °C to increase the annealing time for the sequences 5 and 6. Refer to the Methods for experimental details of the annealing process. ( a ) Fermi surface evolution during the annealing process. ( b – d ) Band structure evolution for the momentum cuts across Γ ( b ), M2 ( c ) and M3 ( d ). The location of the three cuts are the same as shown in Fig. 3e . The band structures shown here are second derivatives of the original images with respect to energy. ( e ) Band structure (original data) of the annealed double-layer FeSe/SrTiO 3 film (corresponding to the sequence 6) measured along cut 2 across M2 at 23 K (left panel) and 75 K (right panel). The photoemission images are divided by the corresponding Fermi distribution function to highlight opening or closing of an energy gap. ( f ) Corresponding symmetrized EDCs on the Fermi momentum measured at different temperatures. Full size image Figure 5 shows the Fermi surface and band structure evolution of the double-layer FeSe/SrTiO 3 film (sample #2) under another annealing condition to gradually increase the annealing temperature. To avoid redundancy, we started with the initial sample that is already annealed for a couple of cycles at lower temperatures and then annealed at 350 °C (sequence 1 for sample #2). It shows dominant N phase features, and also some signatures of the S phase. With further annealing, the bands corresponding to the N phase (N1, N2 and N3 bands) get weaker while the S phase bands (S1, S2 and S3 bands) get stronger. When it comes to the sequences 5 and 6, the N phase disappears and the measured electronic structure is dominated by the pure S phase. Such a Fermi surface and band structure evolution follows a rather similar trend as that for the single-layer FeSe/SrTiO 3 sample [8] . It appears that higher annealing temperature is more effective in giving rise to the transition from the N phase to the S phase, although the annealing time is much shorter than that used for the sample #1 ( Fig. 4 ). Figure 5e shows the band structure measured at different temperatures along the M2 cut for the sequence 6. The corresponding symmetrized EDCs measured at different temperatures on the Fermi momentum are shown in Fig. 5f . One can see a sharp coherence peak, and a clear gap opening at low temperature with a size of 13.5 meV, which gets closed near 55 K. These observations are similar to that observed in the single-layer FeSe/SrTiO 3 film [7] , [8] , [9] , which indicate that the sample for the sequence 6 is superconducting. During the annealing of the double-layer FeSe/SrTiO 3 films, we realized that the situation can be more complicated than annealing the single-layer FeSe/SrTiO 3 films. In addition to the doping effect that is involved, there is also a possibility of FeSe evaporation during the annealing process. For the single-layer FeSe/SrTiO 3 film, we can always probe the electronic structure of the single-layer FeSe film because the bare SrTiO 3 substrate does not contribute an obvious signal [8] , [9] even if some portion of the FeSe layer is evaporated. However, in the case of the double-layer FeSe/SrTiO 3 film, there is a possibility that the top layer may evaporate and the sample may gradually become mixed with double-layer and single-layer regions. To examine this possibility, we checked the FeSe/SrTiO 3 films using STM before and after annealing under different conditions. As shown in Fig. 6a,b , when the annealing temperature is relatively low (450 °C in this case), after annealing for 15 h, the double-layer region remains nearly intact with a similar occupation ratio before and after annealing. However, as seen from Fig. 6c,d , when the annealing temperature is increased to 500 °C, after annealing for only 3 h, the area of the initial triple-layer region is obviously reduced, and a single-layer region emerges that is absent in the original sample. This indicates that at a high annealing temperature (~500 °C and above), significant FeSe evaporation can occur during the annealing process. 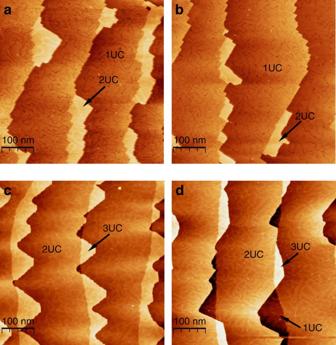Figure 6:  STM topography of FeSe/SrTiO3films before and after being annealed under different conditions. (a) STM image of an as-grown single-layer-dominant FeSe/SrTiO3film. (b) STM image after the sample was annealed at 450 °C for 15 h. The grey areas represent single layer (1UC) while the bright areas represent double layer (2UC), as marked by arrows. (c) STM image of an as-grown double-layer-dominant FeSe/SrTiO3film. (d) Its corresponding STM image after being annealed at 500 °C for 3 h. In this case, the dark region represents the single-layer area (1UC), grey regions represent the double-layer area (2UC) and the bright region represents the triple-layer area, as marked by arrows. Before annealing, double-layer regions dominate with a small amount of triple-layer regions. After annealing at 500 °C for 3 h, the area of the initial triple-layer regions is reduced, and single-layer regions emerge that are absent in the original sample before annealing. Note that, in both samples, the field of view taken before and after the annealing are not exactly on the same area. Figure 6:  STM topography of FeSe/SrTiO 3 films before and after being annealed under different conditions. ( a ) STM image of an as-grown single-layer-dominant FeSe/SrTiO 3 film. ( b ) STM image after the sample was annealed at 450 °C for 15 h. The grey areas represent single layer (1UC) while the bright areas represent double layer (2UC), as marked by arrows. ( c ) STM image of an as-grown double-layer-dominant FeSe/SrTiO 3 film. ( d ) Its corresponding STM image after being annealed at 500 °C for 3 h. In this case, the dark region represents the single-layer area (1UC), grey regions represent the double-layer area (2UC) and the bright region represents the triple-layer area, as marked by arrows. Before annealing, double-layer regions dominate with a small amount of triple-layer regions. After annealing at 500 °C for 3 h, the area of the initial triple-layer regions is reduced, and single-layer regions emerge that are absent in the original sample before annealing. Note that, in both samples, the field of view taken before and after the annealing are not exactly on the same area. Full size image On the basis of the STM results, we intentionally chose the annealing temperature of 350 °C for the sample #1 of the double-layer FeSe/SrTiO 3 film ( Fig. 4 ). Since it is well below 450 °C used in the STM experiment ( Fig. 6a,b ), the FeSe evaporation can be minimized so that it keeps its double-layer structure during the annealing process. One may argue whether some areas may still become single-layer due to the long annealing time in spite of a low annealing temperature, and whether the signal of the observed S phase may come from the exposed single-layer area, instead of an intrinsic property of the double-layer area. Although we cannot completely rule out this possibility, we believe it is highly unlikely because, if we have single-layer areas present, from our experience of annealing the single-layer FeSe/SrTiO 3 samples [8] , [22] , these single-layer areas should already become superconducting under the annealing conditions we used. This is not consistent with our observation of the broad photoemission spectra and an insulating gap in the S phase ( Fig. 4f ). On the other hand, although we observed a complete transformation of the N phase into the S phase and even the appearance of superconductivity in the sample #2 of the double-layer FeSe/SrTiO 3 film ( Fig. 5 ), from the STM results ( Fig. 6c,d ), it is highly likely that this is due to the evaporation of the top FeSe layer that results in the formation of the single-layer FeSe regions during the annealing process. In other words, these observations reflect the behaviours of the single-layer FeSe/SrTiO 3 film, instead of the double-layer FeSe/SrTiO 3 film that we intended to probe. The above results clearly indicate that the double-layer FeSe/SrTiO 3 film behaves quite differently from the single-layer case in that it is much harder to get doped. Under the same annealing condition when the N phase in the as-prepared single-layer FeSe/SrTiO 3 film is completely transformed into a pure S phase and becomes superconducting, the double-layer film remains mainly in the N phase ( Fig. 3 ). Even after an enhanced annealing by extending the annealing time ( Fig. 4 ), it only reached an early stage of the transformation where the S phase starts to emerge and has a low doping. The complete transformation from the N phase to the S phase requires to further enhance the annealing condition by elevating the annealing temperature, as carried out on the sample #2. However, it is complicated by the possible FeSe evaporation so that it is hard to probe the intrinsic doping evolution of the double-layer FeSe/SrTiO 3 film. The present results of annealing the double-layer FeSe/SrTiO 3 film provide an important insight on the origin of superconductivity in the FeSe/SrTiO 3 films. It has been a prominent issue on where the superconductivity in the single-layer FeSe/SrTiO 3 film originates: from the FeSe layer alone, or the SrTiO 3 substrate or the interface between the SrTiO 3 substrate and the FeSe layer. The dichotomy between the single-layer and double-layer FeSe/SrTiO 3 films makes it clear that the superconductivity cannot originate from the FeSe layer alone. If the superconductivity comes only from the FeSe layer, one would expect that the double-layer FeSe/SrTiO 3 film, especially the top FeSe layer of the double-layer film, would behave similarly like the single-layer FeSe/SrTiO 3 film to become superconducting under the same annealing condition. This result, together with the observation of the markedly different behaviours between the FeSe films grown on graphene [21] and on the SrTiO 3 substrate [6] , point to the significant role of the interface in giving rise to the superconductivity in the FeSe/SrTiO 3 films. The present work on the double-layer FeSe/SrTiO 3 film, as well as that on the single-layer FeSe/SrTiO 3 film [8] , [22] , clearly indicates the essential role of the carrier doping on the superconductivity in the FeSe/SrTiO 3 films, such as, superconductivity occurs only when an appropriate amount of doping is introduced at the interface. The dichotomy of annealing the single-layer and double-layer FeSe/SrTiO 3 films provides further information on the doping mechanism of the FeSe/SrTiO 3 films. First, our observation of the pure N phase in the as-prepared single-layer and double-layer FeSe/SrTiO 3 films indicate that, even when the SrTiO 3 substrate is metallic after the heat treatment at a high temperature accompanied by Se flushing [6] , the FeSe/SrTiO 3 films are not automatically doped in the preparation stage at a relatively low temperature. It is clear that the carrier doping is realized at a late stage when the sample is vacuum annealed at a relatively higher tempetaure [6] , [8] . The pure N phase for the single-layer and double-layer FeSe/SrTiO 3 films was not observed before [9] probably because their preparation temperature is higher than that used in our samples. Second, the present study provides a clear clue on the origin of the carrier doping. As proposed before, there are two possibilities of carrier doping in the vacuum annealing process of the FeSe/SrTiO 3 films. One is the evaporation of Se or formation of the Se vacancies in the FeSe films, while the other is the formation of oxygen vacancies near the SrTiO 3 surface [7] , [8] , [9] . Recent STM measurements on a vacuum-annealed single-layer FeSe/SrTiO 3 film found that [24] , in the as-prepared FeSe film, there are some extra Se adatoms on the surface, and the sample is insulating. In the initial stage of annealing, these extra Se adatoms are gradually removed, and further annealing leads to the formation of Se vacancies. The annealing process gives rise to an insulator–superconductor transition that is in agreement with our ARPES measurements [22] . If the doping process involves only the FeSe film itself, like possible removal of excess Se or formation of Se vacancies, one would expect similar behaviour between the single-layer and double-layer FeSe/SrTiO 3 films under the same annealing conditions, if we consider the effect of the interaction between the top and bottom layers is weak on the doping process. This is apparently not consistent with the markedly different annealing behaviours observed between the single-layer and double-layer FeSe/SrTiO 3 films ( Fig. 3 ). The present results make it clear that the doping process does not involve the FeSe films alone, such as, the evaporation of Se during annealing is not a dominant factor in carrier doping. Recent theoretical calculations also suggest that Se vacancies behave like hole dopants rather than electron dopants [25] . Instead, the SrTiO 3 substrate and the interface between the FeSe and SrTiO 3 must play a major role in the doping process. The dichotomy between the single-layer and double-layer FeSe/SrTiO 3 films can be naturally understood when the carrier doping is realized by the charge transfer from the SrTiO 3 surface. It has been reported that a two-dimensional (2D) electron gas can be formed on the SrTiO 3 (001) surface even when it is annealed in vacuum at a rather low temperature (~300 °C) [26] . As shown before, only when the S phase is formed and the doping level of the S phase exceeds a critical value (~0.089 electrons per Fe) can it become superconducting [22] . In the single-layer FeSe/SrTiO 3 film, all the transferred charge from the SrTiO 3 surface can be taken by the sole FeSe layer, and superconductivity is observed in the doping range over 0.089 electrons per Fe [8] , [22] . However, when it comes to the double-layer or multiple-layer FeSe/SrTiO 3 films, the same charge carriers from the SrTiO 3 surface will be shared by all the FeSe layers, rendering the doping of the bottom FeSe layer much reduced. Here one question arises as to how the charge carriers will be distributed among multiple FeSe layers and how much is left in the bottom layer. The extreme case one may expect is that all the carriers remain confined only near the interface between the SrTiO 3 surface and the bottom FeSe layer. If this is the case, in Figs 3 and 4 , one would expect that the bottom layer of the double-layer FeSe/SrTiO 3 film is completely transformed into the S phase and becomes superconducting, like in the single-layer FeSe/SrTiO 3 film. The top FeSe layer may also become superconducting due to the proximity effect of the superconducting bottom layer. With the photoemission probe depth on the order of 5~10 Å at the photon energy we used (21.2 eV), it is possible to see both layers that gives a mixed signal from the superconducting bottom layer and the undoped top layer. This is apparently not consistent with the measured results in Figs 3 and 4 , where the signal is dominated by the N phase. Although we observed some signal from the S phase after annealing, it shows an insulating behaviour instead of a superconducting behaviour as expected. It is therefore more plausible that the carriers from the charge reservoir of the SrTiO 3 surface is spread over all FeSe layers, but in an uneven manner: the FeSe layer closer to the interface gets more doped while the FeSe layer farther away from the interface gets less doped. This can explain why the double-layer or multiple-layer FeSe films are harder to get doped to become superconducting, because the spread of the charge carriers over all the FeSe layers makes the doping on the bottom FeSe layer low that is not sufficient to reach the critical doping level as required in realizing superconductivity [8] , [22] . One may further expect that the thicker the FeSe/SrTiO 3 film is, the harder it is to dope, and the easier it is to stay as an N phase. Because ARPES and STM are surface-sensitive techniques that probe mainly the top one or two layers that are least doped, this explains why one sees a robust N phase in the double-layer film here and in the multiple-layer FeSe/SrTiO 3 films [9] . The present work provides clues on understanding a number of issues associated with the superconductivity in the FeSe/SrTiO 3 films and the bulk FeSe sample. It sheds light on the nature of the parent compound for the bulk FeSe superconductor. It is clear that the molecular beam epitaxy (MBE)-grown FeSe/SrTiO 3 films behave differently from the bulk FeSe in that the FeSe/SrTiO 3 films exhibit a possible magnetic state (N phase) that is absent in the bulk FeSe sample. Moreover, the multi-layer FeSe/SrTiO 3 films do not seem to recover to be a bulk superconductor even up to 50 layers [9] . The difference can be attributed to the delicate variation in the sample composition. In the MBE-grown FeSe/SrTiO 3 films, the atomic control of the composition makes it possible to prepare FeSe 1+ x or FeSe 1− x films that are nearly perfect for the Fe ordering, although there may be Se adatoms or Se vacancies formation [24] . On the other hand, for the bulk Fe 1+ x Se superconductor, slight excess Fe is inevitable and necessary for stabilizing the crystal structure [4] , [27] while iron vacancies can be formed in the nano-form of the Fe 1− x Se compounds [28] . It has been demonstrated that the property and superconductivity of the FeSe system is very sensitive to its composition and stoichiometry [29] . The observation of the possible magnetic N phase in the as-prepared FeSe/SrTiO 3 films, and its transformation into the S phase and becoming superconducting via doping, make it clear that this N phase, instead of FeTe commonly believed [30] , can be the parent compound for the family of the FeSe superconductor. On the other hand, the different behaviours among single-layer, double-layer and multi-layer FeSe/SrTiO 3 films, such as their different transition temperatures ( Fig. 2i ), indicate that some factors other than composition must come into play. The markedly different behaviours between the FeSe/SrTiO 3 and FeSe/graphene [21] films indicate that the substrate must play an important role. In FeSe/SrTiO 3 films, we believe there are two important factors that may account for the layer-dependent behaviours. The first is the tensile strain. When the FeSe film is deposited on the SrTiO 3 substrate, because the lattice constant of SrTiO 3 (3.905 Å) is larger than the bulk FeSe (3.76 Å), the FeSe films are under a tensile stress. When the FeSe films get elongated, one may expect the electron correlation gets stronger and the possible magnetic ordering gets enhanced [17] . In this case, the single-layer FeSe film would get affected the most. With the increase of the FeSe layers, the tensile stress on the top FeSe layers will be gradually relaxed in the multi-layer FeSe/SrTiO 3 films. The second factor is the dimensionality. It can be expected that the 2D system exhibits stronger electron correlation than the three-dimensional (3D) counterpart mainly because the electron-hopping term is reduced in two dimensions due to less coordination numbers. The single-layer FeSe film exhibits the strongest 2D effect that it should exhibit a strong electron correlation. With the increase of the FeSe layers, the system gradually transforms from 2D to 3D accompanied with a decrease of electron correlation. Combining the effect of both the tensile strain and the dimensionality, it is expected that the single-layer FeSe/SrTiO 3 film should have the strongest electron correlation that may be related to its highest possible magnetic transition temperature. The effect will get weaker with the increasing FeSe layers, but it is a gradual process that may extend to multi-layer FeSe/SrTiO 3 films, as seen in Fig. 2i . We note here that, while doping and electron correlation are important factors in affecting superconductivity in the FeSe/SrTiO 3 films, other effects, such as the interaction between the FeSe film and the SrTiO 3 substrate, also need to be considered in understanding the T c enhancement in the single-layer FeSe/SrTiO 3 films. First-principle calculations indicate that both the single-layer and double-layer FeSe/SrTiO 3 films behave like slightly doped semiconductors, with a collinear antiferromagnetic order on the Fe ions [10] . It was further shown that the SrTiO 3 substrate-induced tensile strain tends to stabilize the collinear antiferromagnetic state in FeSe thin film by enhancing the next-nearest-neighbour super-exchange antiferromagnetic interaction bridged through the Se atoms [17] . The calculated Fermi surface considering the collinear antiferromagnetic order is consistent with experimental observations that the hole-like Fermi surface sheets near Γ disappear [17] . In the presence of constrained magnetization, it was also shown that the observed Fermi surface can be described by the checkerboard antiferromagnetic spin pattern [12] , [13] . In this case, it was found that the system has a considerable charge transfer from SrTiO 3 substrate to the FeSe layer, and so has a self-constructed electric field. The disappearance of the Fermi surface around the Γ point can also be explained by the antiferromagnetic checkerboard phase with charge doping and electric field effects [13] . These calculations all involve antiferromagnetic order, and are overall consistent with experimental observations. We note that, the ARPES results are only suggestive that the N phase of the FeSe/SrTiO 3 films is possibly magnetic and further direct evidence is needed to pin down on its magnetic nature. The present work points to a new possibility in inducing or enhancing superconductivity in the double-layer or multiple-layer FeSe/SrTiO 3 films. We have clearly shown that the electronic evolution of the double-layer FeSe/SrTiO 3 film shows a tendency to follow a similar route as in the single-layer film (emergence of the S phase with annealing, Fig. 4 ). It is now clear that the difficulty in achieving a metallic or superconducting state in the double-layer and multiple-layer FeSe/SrTiO 3 films lies in how to effectively dope the FeSe layers into an appropriate doping level. As it is common in the high-temperature cuprate superconductors that the existence of multiple-CuO 2 planes in one unit cell may exhibit higher superconducting transition temperature than its single-layer counterparts [31] , it is interesting to explore whether the double-layer FeSe/SrTiO 3 film, or the multiple-layer FeSe/SrTiO 3 films, may become superconducting and possess even higher T c than the single-layer film if doped properly. To enhance the doping in the double-layer and multiple-layer FeSe/SrTiO 3 films, and to overcome the complication of the FeSe evaporation, one has to take a different approach from the present simple annealing process. This can be realized by either substitution within the FeSe films or chemical deposition on the top of the FeSe surface. This provides an additional handle to tune superconductivity in the FeSe/SrTiO 3 films. It is expected that future study along this line will shed more insight on the origin of high-temperature superconductivity in the FeSe/SrTiO 3 films. The marked difference between the single-layer and double-layer FeSe/SrTiO 3 films also provides a layer-engineering technique to fabricate electronic devices by making metallic, superconducting and insulating components on the same substrate under the same preparation conditions. Preparation of FeSe/SrTiO 3 thin films The single-layer and double-layer FeSe films were grown on SrTiO 3 (001) substrate by the MBE method and were characterized using a scanning tunnelling microscope [6] . To improve the sample quality, the growth procedure usually involves two steps: the first step is to grow the film at a relatively low temperature, and the second step is to anneal the as-prepared sample at a relatively high temperature [6] . For the single-layer FeSe/SrTiO 3 film, it has been shown that the as-prepared film is not superconducting and it becomes superconducting only after it is vacuum annealed at a high temperature [8] . The prepared FeSe/SrTiO 3 films were capped by amorphous Se to protect the samples from the air when transferring the sample out of the MBE chamber into the ARPES annealing and measurement chambers. Post-annealing of FeSe/SrTiO 3 films In this work, we started with the as-prepared FeSe/SrTiO 3 films and annealed it in our own sample annealing chamber that is connected with the ARPES measurement chamber. The sample was first annealed in the annealing chamber at a low temperature (190 °C) to remove the capping layer of amorphous Se. Then it experienced many sequences of annealing in vacuum at various temperatures and for different times. After each annealing, the sample was transferred into the ARPES chamber to measure the band structure, Fermi surface and energy gap. 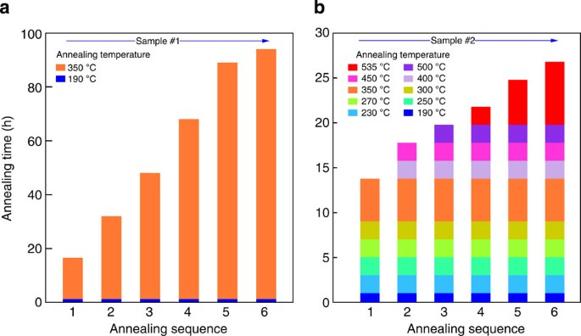Figure 7:  Annealing conditions for two double-layer FeSe/SrTiO3films. (a) The sample #1 was annealed at a relatively low but constant temperature of 350 °C for different times. (b) The sample #2 was annealed at gradually increasing temperatures. The colour bar represents the annealing temperature while the bar height represents the annealing time. The annealing is an accumulative process, such as, for a given sample, the annealing is on top of the previous sequence. For example, for the annealing sequence 1 of sample #1, it means the sample #1 has been annealed first at 190 °C for nearly 1 h, then at 350 °C for nearly 15 h. Figure 7 shows the annealing conditions for two typical as-prepared double-layer FeSe/SrTiO 3 films. Different colours represent different annealing temperatures, and the height of the bar represents the annealing time. For a given sample, the annealing process was carried out sequentially by keeping a constant temperature ( Fig. 7a ) or gradually increasing the annealing temperature ( Fig. 7b ) and time. It therefore produced an accumulative annealing effect to the sample. As shown in Fig. 7a , the sample #1 was annealed six times, denoted as six annealing sequences 1–6. For example, for the annealing sequence 1, the as-prepared sample #1 was first annealed at 190 °C for 1.2 h, mainly to remove the amorphous Se-capping layer, followed by annealing at 350 °C for 15.3 h. For the annealing sequence 6, the sample #1 has been annealed in vacuum altogether at 190 °C for 1.2 h and at 350 °C for an accumulative 92.75 h. For the double-layer FeSe/SrTiO 3 sample #2 ( Fig. 7b ), we show six annealing sequences with different annealing temperatures. To avoid redundancy, we started with the initial sample that was already annealed for a couple of cycles at lower temperatures and then annealed at 350 °C (sequence 1 for sample #2). Till the last sequence 6, the sample #2 was annealed many cycles with the last annealing at 535 °C for 11 h. Figure 7:  Annealing conditions for two double-layer FeSe/SrTiO 3 films. ( a ) The sample #1 was annealed at a relatively low but constant temperature of 350 °C for different times. ( b ) The sample #2 was annealed at gradually increasing temperatures. The colour bar represents the annealing temperature while the bar height represents the annealing time. The annealing is an accumulative process, such as, for a given sample, the annealing is on top of the previous sequence. For example, for the annealing sequence 1 of sample #1, it means the sample #1 has been annealed first at 190 °C for nearly 1 h, then at 350 °C for nearly 15 h. Full size image High-resolution ARPES measurements High-resolution angle-resolved photoemission measurements were carried out on our lab system equipped with a Scienta R4000 electron energy analyzer [32] . We use helium discharge lamp as the light source, which can provide photon energies of hυ =21.218 eV. The energy resolution was set at 10~20 meV for the Fermi surface mapping and band structure measurements, and 4~10 meV for the gap measurements. The angular resolution is 0.3°. The Fermi level ( E F ) is referenced by measuring on the Fermi edge of a clean polycrystalline gold that is electrically connected to the sample. The ARPES measurement was carried out with a base pressure better than 5 × 10 −11 Torr. Sample temperature calibration Since the double-layer FeSe film is grown on the SrTiO 3 substrate, when it is tightened on the sample holder by copper pads, the thermal conductivity of the film becomes poorer than that of the usual cleaved sample, which is directly fixed on the sample holder using silver paste. Therefore, the usual sample temperature sets a low limit to the temperature of the FeSe film. To measure the temperature of the FeSe film more accurately, we mimicked the FeSe film’s situation by gluing a piece of polycrystalline gold foil on the similar SrTiO 3 substrate. By measuring the Fermi level of the gold from our high-resolution laser photoemission, we can measure the temperature of gold on SrTiO 3 from the gold Fermi edge broadening fitted by the Fermi distribution function. Since the Fermi edge width contains a couple of contributions including the temperature broadening, instrumental resolution and cleanliness of gold, the estimated temperature sets an upper limit to the gold temperature, which is close to the temperature of FeSe thin film on SrTiO 3 . We found the temperature measured from this gold reference is higher than the nominal usual sample temperature by ~10 K. The real temperature of the FeSe thin film lies then in between these two temperature limits, nominal sample temperature and gold temperature, with an error bar of ±5 K. How to cite this article : Liu, X. et al. Dichotomy of the electronic structure and superconductivity between single-layer and double-layer FeSe/SrTiO 3 films. Nat. Commun. 5:5047 doi: 10.1038/ncomms6047 (2014).